Structural analysis of human 2′-O-ribose methyltransferases involved in mRNA cap structure formation The 5′ cap of human messenger RNA contains 2′- O -methylation of the first and often second transcribed nucleotide that is important for its processing, translation and stability. Human enzymes that methylate these nucleotides, termed CMTr1 and CMTr2, respectively, have recently been identified. However, the structures of these enzymes and their mechanisms of action remain unknown. In the present study, we solve the crystal structures of the active CMTr1 catalytic domain in complex with a methyl group donor and a capped oligoribonucleotide, thereby revealing the mechanism of specific recognition of capped RNA. This mechanism differs significantly from viral enzymes, thus providing a framework for their specific targeting. Based on the crystal structure of CMTr1, a comparative model of the CMTr2 catalytic domain is generated. This model, together with mutational analysis, leads to the identification of residues involved in RNA and methyl group donor binding. Messenger RNAs (mRNAs) of all eukaryotic organisms and many viral RNAs possess a 5′ cap structure that consists of an N 7 -methylguanosine (m 7 G) linked via an inverted 5′–5′ triphosphate bridge to the 5′-terminal nucleoside of the transcript [1] . This cap0 structure is essential for the cell growth of Saccharomyces cerevisiae [2] and survival of mammalian cells [3] . Cap0 is critical for mRNA interactions with many nuclear and cytoplasmic proteins and plays multiple roles in gene expression, including the enhancement of RNA stability, splicing, nucleocytoplasmic transport and translation initiation [4] , [5] . In higher eukaryotes, mRNA and small nuclear RNA (snRNA) 5′ ends are further modified by methylation of the ribose on the first and second transcribed nucleosides (that is, cap1 and cap2, respectively) [6] . In humans, cap0 and cap1 methylations are present on all mRNA molecules, whereas approximately half of the capped and polyadenylated RNA molecules contain cap2 methylation [7] . The U1, U2, U4 and U5 snRNAs are methylated at the first two positions [8] . Cap1 and cap2 methylations in U2 snRNA are required for spliceosomal E complex formation and consequently for efficient pre-mRNA splicing [9] . Uncapped RNAs, such as nascent viral transcripts, may be detected as ‘non-self’ by the host cell, triggering an antiviral innate immune response through the production of interferons [10] . Therefore, many viruses that replicate in the cytoplasm of eukaryotes have evolved 2′- O -methyltransferases (2′- O -MTases) to autonomously modify their mRNAs. Although the RNA cap structures that originate from human and viral enzymes are identical, the structure and catalytic mechanisms of the virus-encoded enzymes involved in the synthesis of the RNA cap structure are different from those of host cells. As a consequence, these pathogenic cap-forming enzymes are potential targets for antimicrobial drugs (as reviewed in ref. 11 ). Several potent inhibitors of viral cap1 MTases were recently identified, but their specificity and lack of toxicity (for example, the absence of interactions with human enzymes) remain to be established [12] . To date, numerous high-resolution structures of viral RNA capping enzymes have been determined, but only a few of them represent complexes with RNA and shed light on specific cap recognition. This is partially because the availability of 5′-capped RNA substrates with a defined and appropriate length has remained an important bottleneck. A structure of vaccinia virus cap1 MTase VP39 has been solved as a ternary complex with S -adenosyl- L -homocysteine (SAH) and a capped RNA [13] . A number of structures of cap1 MTases from flaviviruses were determined with various cap analogues, revealing the structure of the cap-binding pocket [14] , [15] . The development of compounds that inhibit viral cap1 MTases has been, however, greatly limited by the lack of structural information about the corresponding human enzymes that must not be inhibited by the virus-specific drugs. Genes that encode the human cap1 and cap2 MTases (that is, CMTr1 and CMTr2) have been only recently discovered [16] , [17] , enabling detailed biochemical and structural characterization of their products. In the present study, we report crystal structures of an isolated, functionally active CMTr1 catalytic domain in several forms, including a complex with a capped oligoribonucleotide (m 7 GpppGAUC). Furthermore, a model of the CMTr2 catalytic domain bound to its target is presented. These structures reveal key differences in cap binding by human and viral enzymes, providing a framework for the search for viral cap MTase-specific inhibitors. Deletion analysis of cap MTases To understand the contribution of individual domains to the function of CMTr1 and CMTr2, we created deletion variants of each protein. For CMTr1, one of the variants (CMTr1 1–550 ) contained the catalytic Rossmann-fold MTase (RFM) domain, G-patch and nuclear localization signal, and the other variant (CMTr1 550–835 ) contained the remaining carboxy-terminal part that comprises the guanylyltransferase-like and WW domains ( Fig. 1a ). CMTr2 was also divided into two parts: the amino-terminal part with the catalytic RFM domain (CMTr2 1–430 ) and the C-terminal part with the non-catalytic RFM domain (CMTr2 430–770 ) ( Fig. 2a ). CMTr1 1–550 is able to bind a cap0-RNA substrate and methylate it, and the C-terminal guanylyltransferase-like domain of CMTr1 is not essential but contributes to the MTase activity of this protein ( Fig. 3 ). The single domains of CMTr2 do not bind the substrate and do not exhibit any cap MTase activity alone or when mixed together as separately purified chains. Thus, CMTr2 requires both RFM domains in a single polypeptide chain for substrate binding and methylation. 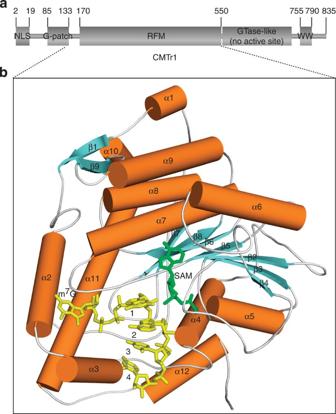Figure 1: Crystal structure of the catalytic MTase domain of CMTr1. (a) Domain composition of full-length CMTr1. The dashed lines indicate the region of the protein (CMTr1126–550) present in the crystal structure. The domain boundaries are indicated with residue numbers. (b) Crystal structure of CMTr1126–550in complex with capped oligoribonucleotide (m7GpppGAUC; coloured yellow) and SAM (green). Helices are shown in orange, β-strands are shown in blue and loops are shown in white. Figure 1: Crystal structure of the catalytic MTase domain of CMTr1. ( a ) Domain composition of full-length CMTr1. The dashed lines indicate the region of the protein (CMTr1 126–550 ) present in the crystal structure. The domain boundaries are indicated with residue numbers. ( b ) Crystal structure of CMTr1 126–550 in complex with capped oligoribonucleotide (m 7 GpppGAUC; coloured yellow) and SAM (green). Helices are shown in orange, β-strands are shown in blue and loops are shown in white. 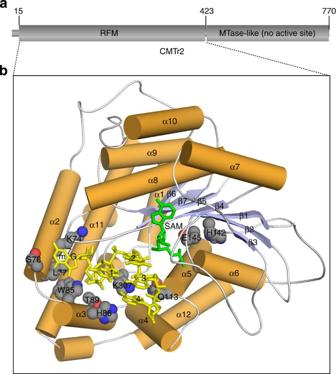Figure 2: Homology model of CMTr21–423. (a) Domain composition of CMTr2. The dashed lines indicate a part of the protein that was modelled based on the CMTr1126–550crystal structure. The domain boundaries are indicated with residue numbers. (b) Homology model of the catalytic domain of CMTr2 in complex with capped oligoribonucleotide (m7GpppGGAA) and SAM. m7GpppGGAA and SAM are coloured yellow and green, respectively. Helices are shown in orange, β-strands are shown in blue and loops are shown in white. Residues that were studied in directed mutagenesis experiments are shown in gray spheres. Full size image Figure 2: Homology model of CMTr2 1–423 . ( a ) Domain composition of CMTr2. The dashed lines indicate a part of the protein that was modelled based on the CMTr1 126–550 crystal structure. The domain boundaries are indicated with residue numbers. ( b ) Homology model of the catalytic domain of CMTr2 in complex with capped oligoribonucleotide (m 7 GpppGGAA) and SAM. m 7 GpppGGAA and SAM are coloured yellow and green, respectively. Helices are shown in orange, β-strands are shown in blue and loops are shown in white. Residues that were studied in directed mutagenesis experiments are shown in gray spheres. 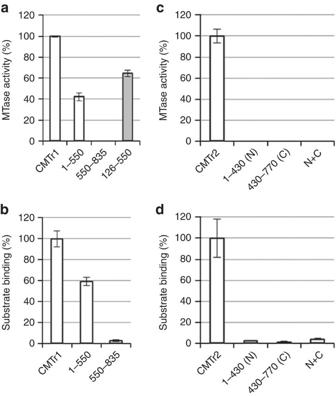Figure 3: Biochemical characterization of CMTr1 and CMTr2 and their fragments. The analysis was performed for full-length proteins and deletion variants of CMTr1 (a,b) and CMTr2 (c,d). The proteins were overexpressed in and isolated from HEK 293 cells (white bars) orE.coli(grey bar). Protein variant CMTr1 126–550 was expressed from crystallization construct. (a,c) MTase activity.In vitrotranscribed RNA-GG molecules with a32P-labelled cap0 (a) or cap01 (c) structure were incubated with the indicated enzymes in the presence of SAM. Product RNA was digested with nuclease P1 (a) or RNase T2 (c) and purified by phenol/chloroform extraction and ethanol precipitation. The digestion products were resolved on 21% polyacrylamide/8 M urea gel and quantified after autoradiographic visualization. (b,d) Substrate binding.In vitrotranscribed RNA-GG molecules with a32P-labelled cap0 (b) or cap01 (d) structure were incubated with the indicated enzymes in the presence of SAH (the product of SAM demethylation) and uncapped, competitor RNA to detect specific substrate binding. After 30 min incubation, the samples were filtered through a nitrocellulose membrane and washed with reaction buffer. RNA bound to membrane-attached proteins was visualized by autoradiography and quantified. The signal from the negative control (that is, the sample with BAP protein) was subtracted from the signal from samples with cap MTases. The analyses were performed in triplicate. The relative activity/binding compared with the full-length enzyme (set at 100%) and s.d. values are shown. Full size image Figure 3: Biochemical characterization of CMTr1 and CMTr2 and their fragments. The analysis was performed for full-length proteins and deletion variants of CMTr1 ( a , b ) and CMTr2 ( c , d ). The proteins were overexpressed in and isolated from HEK 293 cells (white bars) or E . coli (grey bar). Protein variant CMTr1 126–550 was expressed from crystallization construct. ( a , c ) MTase activity. In vitro transcribed RNA-GG molecules with a 32 P-labelled cap0 ( a ) or cap01 ( c ) structure were incubated with the indicated enzymes in the presence of SAM. Product RNA was digested with nuclease P1 ( a ) or RNase T2 ( c ) and purified by phenol/chloroform extraction and ethanol precipitation. The digestion products were resolved on 21% polyacrylamide/8 M urea gel and quantified after autoradiographic visualization. ( b , d ) Substrate binding. In vitro transcribed RNA-GG molecules with a 32 P-labelled cap0 ( b ) or cap01 ( d ) structure were incubated with the indicated enzymes in the presence of SAH (the product of SAM demethylation) and uncapped, competitor RNA to detect specific substrate binding. After 30 min incubation, the samples were filtered through a nitrocellulose membrane and washed with reaction buffer. RNA bound to membrane-attached proteins was visualized by autoradiography and quantified. The signal from the negative control (that is, the sample with BAP protein) was subtracted from the signal from samples with cap MTases. The analyses were performed in triplicate. The relative activity/binding compared with the full-length enzyme (set at 100%) and s.d. values are shown. Full size image CMTr1 catalytic domain structure To elucidate the mechanism of cap recognition and methylation by CMTr1, we solved its crystal structure in complex with ligands. We expressed several deletion mutants in Escherichia coli and finally identified a stable CMTr1 variant that comprised a catalytic domain (residues 126–550; described in detail in the Supplementary Methods ). The enzymatic activity of CMTr1 126–550 was confirmed in vitro ( Supplementary Fig. S1 ); consequently, this protein variant was used in the crystallization trials. We determined three crystal structures of the catalytic RFM domain of CMTr1: (i) an unliganded form at 2.35 Å resolution, (ii) a ternary complex with cofactor S -adenosyl methionine (SAM) and an mRNA cap analogue (m 7 GpppG) at 1.9 Å resolution and (iii) a complex with SAM and a capped oligoribonucleotide at 2.7 Å resolution ( Table 1 ). The three structures belong to space groups I 422 (i), P 2 1 (ii) and P 1 with two protein molecules in the asymmetric unit (iii) and together comprise four independent determinations of the protein structure. All four protein models are nearly identical and can be superimposed with a root mean squared deviation (r.m.s.d.) between 0.3 Å (structure (ii) versus (iii), 367 pairs of C-α atoms) and 0.7 Å (structure (i) versus (iii), 336 pairs of C-α atoms). The structural differences are limited to minor conformational changes of several loops upon substrate binding ( Supplementary Fig. S2a ). Complex structure (iii) with a capped oligoribonucleotide is shown in Fig. 1b . Table 1 Statistics for SAD (SeMet) structure and molecular replacement. Full size table The catalytic RFM domain of CMTr1 adopts the eponymous Rossmann-like fold [18] . The core of the domain comprises a characteristic β-sheet with seven strands surrounded by six α-helices (that is, a structure conserved in nearly all members of the RFM superfamily). The peripheral extensions, both at the N- and C-termini, resemble the structures found in other cap-modifying MTases, including vaccinia virus VP39 protein that acts as a cap1 MTase [13] , and a bifunctional cap0/cap1 MTase domain of flaviviruses [19] . In fact, viral cap1 MTases are the closest structural matches of the CMTr1 catalytic domain according to the DALI server [20] . Substrate and cofactor binding by the CMTr1 catalytic domain In structures (ii) and (iii), we observed well-defined electron densities for the ligands ( Supplementary Fig. S3 ). For both complexes, the SAM cofactor is bound in a deep pocket located at the edge of the central β-sheet between strands 2, 3 and 4 ( Fig. 1b ). SAM binding is very similar to other RFM MTases, such as the NS5 protein from dengue virus [21] and VP39 protein from vaccinia virus [13] . In the structure of CMTr1 126–550 in complex with SAM and a capped oligoribonucleotide substrate (structure (iii)), the nucleic acid adopts an L shape, with the methylated guanosine (m 7 G) accommodated in a deep pocket, and the methylatable nucleotide 1 located at the bend of the substrate molecule ( Fig. 1b ). The remainder of the mRNA exits from the binding site through a positively charged channel on the protein surface ( Fig. 4a and Supplementary Fig. S4a,b ). With the exception of the m 7 G residue, the interactions occur between the protein and phosphodiester backbone of the nucleic acid. The lack of contacts between the bases of the RNA and CMTr1 protein suggests that substrate binding and methylation are sequence-independent ( Fig. 4c ). 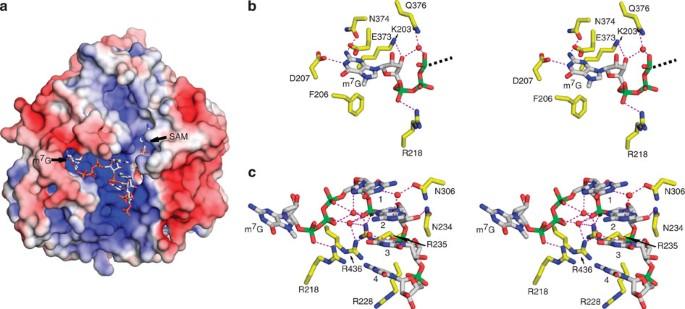Figure 4: Substrate and cofactor binding by CMTr1126–550 (a) Surface representation of CMTr1126–550with electrostatic potential (±5 kT/e, red-negative; blue-positive). Capped oligoribonucleotide and SAM are shown in stick representation. (b) Stereo view of the interactions between the protein and m7Gppp. The remainder of the RNA (four ribonucleotide residues) is omitted for clarity. (c) Stereo view of capped oligoribonucleotide binding. Water molecules that mediate the binding are shown as small red spheres. Figure 4: Substrate and cofactor binding by CMTr1 126–550 ( a ) Surface representation of CMTr1 126–550 with electrostatic potential (±5 kT/e, red-negative; blue-positive). Capped oligoribonucleotide and SAM are shown in stick representation. ( b ) Stereo view of the interactions between the protein and m 7 Gppp. The remainder of the RNA (four ribonucleotide residues) is omitted for clarity. ( c ) Stereo view of capped oligoribonucleotide binding. Water molecules that mediate the binding are shown as small red spheres. Full size image m 7 G binding and conformation are essentially identical between the structures of CMTr1 with the cap analogue (structure (ii)) and capped oligoribonucleotide (structure (iii)), but the position of γ-phosphate differs. This likely results from the fact that the first transcribed nucleotide of m 7 GpppG is disordered and not visible in the structure. The bottom of the m 7 G-binding pocket is formed by the side chain of K203, and the amine group of this residue forms a hydrogen bond with the 2′-OH group of the ribose of m 7 G ( Fig. 4b ). The side chain of E373 forms a stacking interaction with the aromatic ring of m 7 G. Additional interactions that stabilize the m 7 G part of the capped oligoribonucleotide are between D207 and N 1 of the m 7 G base and between N374 and N 2 of the base. R218, Q376 and D439 interact with the triphosphate bridge. The importance of the m 7 G moiety for substrate binding and recognition is confirmed by the observation that RNA molecules without 5′ cap guanosine are not methylated by CMTr1, and human cap MTases generally appear to act only on a capped 5′ end of RNA ( Supplementary Fig. S5 ). In structure (iii), the key element that stabilizes the m 7 GpppGAUC substrate is three guanidinium groups of arginine residues 218, 235 and 436, which all form a stacking sandwich that places a cluster of positive charges inside the turn of L-shaped substrate molecule ( Fig. 4c ). The cluster interacts both directly and through water molecules with phosphate groups of the triphosphate linker and nucleotides 2 and 3 of the RNA. An additional residue that stabilizes the RNA backbone is K239, which, together with D364 and K404, forms the active site. The base of nucleotide 1 abuts the surface formed by the main chain of the protein (residues 366–368) and interacts with it through van der Waals contacts. The side chain amide group of N234 forms a hydrogen bond with the 2′-OH group of the ribose of the second transcribed nucleotide. Model of the CMTr2 catalytic domain in complex with RNA To facilitate comparisons between CMTr1 and CMTr2, we built a structural model of the CMTr2 1–423 catalytic domain by comparative modelling, using the CMTr1 126–550 structure as a template ( Fig. 2b ; see Methods for details). According to the model accuracy predictor MetaMQAP [22] , the predicted global root mean squared deviation of the modelled CMTr2 1–423 catalytic domain with respect to the (currently unknown) structure is ~2.3 Å, which indicates good overall quality of the model. This estimation is based on C-α positions; therefore, the atomic details of the model (for example, the conformations of the side chains) should be treated with caution. The RNA substrate of CMTr2 1–423 was also modelled using the comparative approach, with the CMTr1 126–550 substrate structure as the template (see Methods for details). We assumed that the regions that are conserved between CMTr1 126–550 and CMTr2 1–423 should interact with the functionally corresponding nucleotide residues (m 7 G cap and the target ribose) in a very similar way ( Supplementary Fig. S4c–e ). Therefore, the modelling of CMTr2 1–423 substrate RNA involved introducing an insertion of one residue between the 5′–5′ triphosphate and methylated ribose to reflect a register shift between the target of CMTr1 and CMTr2. Substrate and cofactor binding by the CMTr2 catalytic domain Comparisons of the experimentally determined structure of the ternary complex of the CMTr1 126–550 catalytic domain with its RNA substrate, with the corresponding model for the CMTr2 1–423 catalytic domain, reveal an essentially identical active site surrounded by variable residues ( Supplementary Fig. S4e ). The region of identity between the two enzymes spans most of the SAM-binding pocket, the entire active site (including the K-D-K catalytic triad), and the bottom of the cap guanosine-binding pocket. The differences are prominent in the region predicted to accommodate the N 1 residue of the RNA substrate by CMTr2 1–423 , which may explain the different specificities of CMTr1 and CMTr2 (methylation of RNA residue 1 or 2, respectively). The model of the CMTr2 1–423 catalytic domain is not sufficiently accurate to allow us to speculate about the atomic details of N 1 recognition. However, the modelled conformation of RNA agrees well with the experimental information. CMTr2 is able to methylate substrates, regardless of the presence of methylation of the cap guanosine or N 1 ribose [17] . In our model, these methyl groups are exposed to the solvent and are not contacted by the protein. Furthermore, the N 1 residue appears to interact with N 3. During energy minimization, the N 1 conformation converged to form a cis Hoogsteen–Hoogsteen base pair with N 3. In alternative models, N 1 could be forced to flip by 180 degrees and interact with N 3 via the sugar edge. This feature of the model suggests that some base pair combinations in the 5′ end of capped RNAs may be more easily accommodated by the CMTr2 1–423 active site than others, providing a basis for the enzyme substrate specificity. Mutagenesis analysis of CMTr1 and CMTr2 To validate the functional importance of amino-acid residues predicted to be critical for the substrate binding and enzymatic activity of human cap MTases, a mutagenesis analysis was performed. First, two variants of CMTr1 were prepared as controls to validate the method. The alanine substitution of K203 that directly interacts with RNA cap was expected to severely influence the binding and activity of the cap1 MTase. R228 is located in the vicinity of the capped mRNA substrate but does not interact with it, so we expected that R228A substitution would not affect activity or binding. We first analysed the binding and MTase activity of two control variants of CMTr1 with capped oligoribonucleotide (cap0-RNA-GG) as a substrate. As expected, the K203A substitution in CMTr1 strongly affects both the binding and activity of the enzyme, whereas R228A does not ( Fig. 5 ), demonstrating that the method is able to discriminate between the residues that interact with substrate and those that do not. 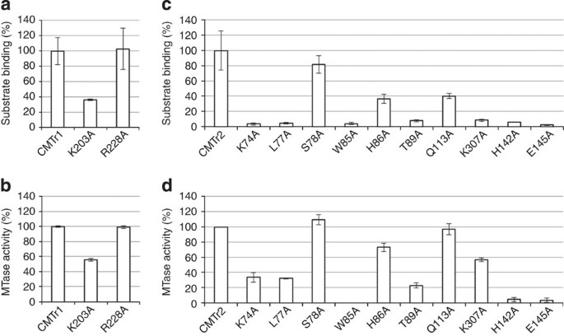Figure 5: MTase activity and RNA binding by CMTr1 and CMTr2 variants with single-residue substitutions. The analysis was performed for full-length wild type and single substitution variants of CMTr1 (a,b) and CMTr2 (c,d). (a,c) Effect of single amino-acid substitutions on MTase activity.In vitrotranscribed RNA-GG molecules with a32P-labelled cap0 (a) or cap01 (c) structure were incubated with the indicated enzymes in the presence of SAM. Product RNA was digested with nuclease P1 (a) or RNase T2 (c) and purified by phenol/chloroform extraction and ethanol precipitation. The digestion products were resolved on 21% polyacrylamide/8 M urea gel and quantified after autoradiographic visualization. (b,d) Effect of single amino-acid substitutions on substrate binding.In vitrotranscribed RNA-GG molecules with a32P-labelled cap0 (b) or cap01 (d) structure were incubated with the indicated enzymes in the presence of SAH. After 30-min incubation, the samples were filtered through a nitrocellulose membrane and washed with a reaction buffer. RNA bound to membrane-attached proteins was visualized by autoradiography and quantified. The signal from the negative control (the sample with the BAP protein) was subtracted from the signal from samples with cap MTases. The analyses were performed in triplicate. The relative activity/binding compared with the wild type enzyme (set at 100%) and s.d. values are shown. Figure 5: MTase activity and RNA binding by CMTr1 and CMTr2 variants with single-residue substitutions. The analysis was performed for full-length wild type and single substitution variants of CMTr1 ( a , b ) and CMTr2 ( c , d ). ( a , c ) Effect of single amino-acid substitutions on MTase activity. In vitro transcribed RNA-GG molecules with a 32 P-labelled cap0 ( a ) or cap01 ( c ) structure were incubated with the indicated enzymes in the presence of SAM. Product RNA was digested with nuclease P1 ( a ) or RNase T2 ( c ) and purified by phenol/chloroform extraction and ethanol precipitation. The digestion products were resolved on 21% polyacrylamide/8 M urea gel and quantified after autoradiographic visualization. ( b , d ) Effect of single amino-acid substitutions on substrate binding. In vitro transcribed RNA-GG molecules with a 32 P-labelled cap0 ( b ) or cap01 ( d ) structure were incubated with the indicated enzymes in the presence of SAH. After 30-min incubation, the samples were filtered through a nitrocellulose membrane and washed with a reaction buffer. RNA bound to membrane-attached proteins was visualized by autoradiography and quantified. The signal from the negative control (the sample with the BAP protein) was subtracted from the signal from samples with cap MTases. The analyses were performed in triplicate. The relative activity/binding compared with the wild type enzyme (set at 100%) and s.d. values are shown. Full size image We then used an analogous approach for CMTr2 studies. We selected 10 amino-acid residues located either in the conserved part of the active site (common to CMTr1 and CMTr2) or immediately outside of it ( Fig. 2b ). K74 in CMTr2, corresponding to K203 in CMTr1, forms the bottom of the cap-binding site, and L77 was predicted to form a side of the cap-binding site. Further selected residues included W85 (which interacts with L77 and the 5′–5′ phosphate linker), T89 (which binds the 5′–5′ phosphate linker), K307 (which interacts with the RNA backbone), H142 and E145 (which are in the SAM-binding motif), and S78, H86 and Q113 (which are located close to the RNA-binding site but do not form any specific interactions). These residues were individually substituted with alanine. As shown in Fig. 5 , the substitutions of each of the selected residues of CMTr2 affect RNA binding. The catalytic activity of CMTr2 is less affected by the substitutions, but the decrease in activity correlates with the reduction of substrate binding. In agreement with the model, alanine substitutions K74A, L77A, W85A, T89A, K307A, H142A and E145A strongly affect both RNA binding and the catalytic activity of the enzyme. The fact that RNA binding is nearly abolished by the substitution of residues predicted to be important for SAM binding but are not in direct contact with RNA, suggests that cofactor binding by CMTr2 is essential for the binding of RNA. The substitutions of residues S78, H86 and Q113 only mildly affect RNA binding and catalysis, so they are not essential for CMTr2 MTase activity. In conclusion, the results obtained for substituted proteins validated the accuracy of the homology model of CMTr2 and corroborated the residues involved in substrate binding. To date, structural information has only been available for viral 2′- O -ribose mRNA MTases from poxviruses and flaviviruses. Our structure of the human CMTr1 catalytic domain is the first example of a structure determined for a cellular enzyme of this type. It is also only the second enzyme of this group (the other is the VP39 protein form vaccinia virus; Protein Data Bank (PDB) ID: 1AV6 (ref. 13 )) for which a structure with a bound capped oligoribonucleotide substrate is available. The two most strongly conserved elements of the cellular, poxviral and flaviviral enzymes are the SAM-binding pocket determining the position of the methyl group donor and the active site determining the position of the target nucleoside [13] , [14] , [23] . Surprisingly, however, cellular and viral enzymes interact with the guanosine cap in very different ways, although the cap-binding site is located in the same region of their structures ( Fig. 6b ). In vaccinia virus VP39 protein (for example, PDB ID:1AV6 (ref. 13 )), guanosine is almost completely buried in a deep pocket sandwiched between two aromatic chains (Y22 and F180) and oriented with its Hoogsteen edge towards the binding pocket’s floor ( Fig. 6c ). VP39 thereby senses the presence of the methyl group of m 7 G [13] , [24] . In structures of the flavivirus MTases bound to a cap analogue (for example, PDB ID: 2P40 (ref. 14 ) and 3EMB [15] ), the m 7 G residue stacks with one aromatic residue (F24), but the binding site is open to the solvent, and interactions between the methyl group and protein are limited. In the structure of the human CMTr1 determined in the present study and in the theoretical model of CMTr2, m 7 G is bound in a deep pocket, but the sugar edge of the nucleoside residue is directed towards the pocket floor, with the methyl group exposed and involved in few interactions with the protein ( Fig. 6d ). Indeed, the activity of CMTr1 does not depend on the methylation of cap guanosine [16] , [17] , [25] . These differences between the human and viral enzymes are important because they provide the basis for the development of cap analogues that can block the viral cap MTases, without inhibiting the human enzymes. Ribose MTases acting on cap are extensively diverged and the complete understanding of evolutionary transitions between different binding modes will require determination of additional structures for other enzymes from this family [17] , [26] . 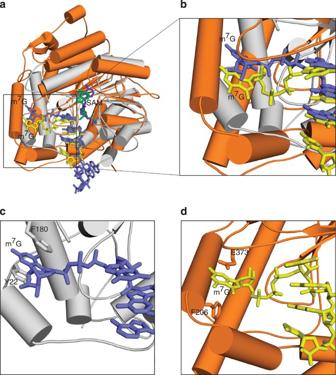Figure 6: Comparison of CMTr1126–550with the viral VP39 enzyme (a) Superimposition of CMTr1126–550substrate complex (orange) on VP39 (PDB ID: 1AV6). (grey) in complex with capped oligoribonucleotide (blue) and SAH (purple). The structures were superimposed using the C-α atoms from the central β-sheet. (b) Close-up view of the m7G-binding pocket. For CMTr1126–550, the protein is coloured orange, and m7G is coloured yellow. For VP39, the protein is coloured grey, and m7G is coloured blue. (c,d) Close-up views of the interactions in m7G binding in VP39 MTase (c) and CMTr1126–550(d). Figure 6: Comparison of CMTr1 126–550 with the viral VP39 enzyme ( a ) Superimposition of CMTr1 126–550 substrate complex (orange) on VP39 (PDB ID: 1AV6). (grey) in complex with capped oligoribonucleotide (blue) and SAH (purple). The structures were superimposed using the C-α atoms from the central β-sheet. ( b ) Close-up view of the m 7 G-binding pocket. For CMTr1 126–550 , the protein is coloured orange, and m 7 G is coloured yellow. For VP39, the protein is coloured grey, and m 7 G is coloured blue. ( c , d ) Close-up views of the interactions in m 7 G binding in VP39 MTase ( c ) and CMTr1 126–550 ( d ). Full size image The common element of the human protein and flaviviral enzymes is the positively charged arginine cluster (formed by R218, R235 and R436 in CMTr1) that stabilizes the triphosphate bridge and phosphate backbone of RNA residues 1 and 2 (refs 23 , 27 , 28 ). Although the core of the catalytic domain of the human and vaccinia enzymes is highly similar ( Fig. 6a ), a prominent difference between the two structures is that the arginine cluster is missing in the latter. In fact, the backbone of the turn of the capped oligoribonucleotide molecule forms very few interactions in the vaccinia MTase–RNA complex. In conclusion, we present the first structural characterization of cellular cap1 and cap2 MTases, revealing a new mode of RNA cap recognition. We also describe similarities and differences with viral enzymes, thus providing a framework for structure-based inhibitor design for those promising drug targets. Eukaryotic overexpression of recombinant proteins CMTr1, CMTr2 and bacterial alkaline phosphatase (BAP) proteins were overexpressed in HEK 293 cells (ATCC) using p3xFLAG-CMV-10 plasmid with an inserted open reading frame of CMTR1 (also known as KIAA0082 , ISG95 , FTSJD2 and HMTR1 ), CMTR2 (also known as AFT , FLJ11171 , FTSJD1 and HMTR2 ), or BAP and jetPEI (Polyplus Transfection) transfection reagent [17] . For recombinant protein purification, cells were resuspended in lysis buffer (50 mM Tris-HCl (pH 7.4), 150 mM NaCl, 1 mM ethylenediaminetetraacetic acid (EDTA), 0.5% Triton X-100, protease inhibitor cocktail for use with mammalian cell and tissue extracts (Sigma)) and after 1 h of incubation centrifuged for 30 min at 20,000 g . Supernatant was incubated with 25 μl ANTI-FLAG M2 Affinity Gel (Sigma-Aldrich) with rotation overnight at 4 °C. Beads were washed following manufacturer recommendations and resuspended in activity assay buffer. Protein samples were run in sodium dodecyl sulfate-polyacrylamide gel electrophoresis to measure the concentration of CMTr1 and BAP in each preparation using densitometry with the use of ImageQuantTL software (GE Healthcare). For CMTr2, the amount of the protein obtained was insufficient for densitometry measurements; therefore, the relative amounts of CMTr2 variants were examined by western blot using monoclonal anti-FLAG M2 antibody produced in mouse (dilution 1:5,000; Sigma-Aldrich) and anti-mouse IgGIRDye 800CW (dilution 1:10,000; LI-COR Biosciences) and analysed with Image Studio software (LI-COR Biosciences). Variants of CMTR1 and CMTR2 were constructed using polymerase chain reaction (PCR). Single amino-acid substitutions were introduced by site-directed mutagenesis. DNA constructs for the expression of deletion variants that contained N-terminal parts of the proteins were prepared by inserting a stop codon after residue 550 for CMTr1 and after residue 430 for CMTr2. The expression of the C-terminal domains was performed using constructs in which the regions that coded residues 2–549 for CMTr1 and 2–429 for CMTr2 were removed. The mutated genes were sequenced and found to contain only the desired changes. Sequences of all primers used in this study are listed in Supplementary Table S1 . Crystallography All of the crystallization trials were performed using the vapor diffusion method at 18 °C with a stock solution of CMTr1 126–550 at a 8–9 mg ml −1 concentration in a buffer that contained 100 mM NaCl, 30 mM Tris-HCl (pH 8.5), 10% glycerol, 0.5 mM EDTA and 3 mM dithiothreitol (DTT). Prior to crystallization, the protein was diluted with water to 4 mg ml −1 and mixed with a well solution at a 1:1 v/v ratio. Crystals of unliganded CMTr1 126–550 were obtained by co-crystallizing the protein with m 7 GpppG and SAM at a final concentration of 0.2 mM for both ligands. The original condition for the crystallization of unliganded CMTr1 126–550 was identified in Index crystallization screen (Hampton Research) and contained 35% Tacsimate (pH 7.0). X-ray diffraction data were collected at beamline 14.1 of BESSY II on a Mar225 CCD detector at 100 K. SeMet protein was crystallized with m 7 GpppG and SAM with both ligands at a concentration of 0.42 mM. The diffraction data from SeMet crystals were collected at 2.9 Å resolution. The structure was solved using single-wavelength anomalous diffraction [29] in Phenix AutoSol module [30] with default parameters. Selenium sites were found by HYSS, experimental phases were calculated in Phaser [31] and density modification with solvent flattening was performed with Resolve. The figure-of-merit after phasing (before solvent modification) was 0.4, and the resulting experimental electron density maps were well defined, allowing the tracing of a model that consisted of residues 141–544 of the protein. The model was then refined against the native data set to 2.35 Å resolution. Although m 7 GpppG and SAM were present in the crystallization mixture, their electron densities were not observed. We refer to this structure as ‘unliganded’ (structure (i)). Different crystal forms of the complex of CMTr1 126–550 with m 7 GpppG and a methyl group donor were obtained by increasing the ligand concentrations in the co-crystallization mixture to 0.85 and 1.71 mM, respectively. They were grown in 30% PEG 3350, 100 mM Bis-Tris (pH 6.5) and 100 mM NaBr as an additive. The structure was solved by molecular replacement using Phaser with a previously obtained unliganded structure as the search model and was refined to a resolution of 1.9 Å (structure (ii); Table 1 ). Crystals of the complex of CMTr1 126–550 with m 7 GpppGAUC and SAM were obtained as a result co-crystallizing the protein with both ligands at concentrations of 0.85 and 1.71 mM, respectively. The crystals were grown in 30% PEG 3350, 100 mM Bis-Tris (pH 6.5) and 100 mM NaBr as an additive. The structure was solved by molecular replacement using Phaser with the structure of CMTr1 126–550 complex with m 7 GpppG and SAM as a search model and refined to a resolution of 2.7 Å (structure (iii); Table 1 ). The asymmetric unit contains two copies of the protein complex. In one copy, the electron densities for the capped oligoribonucleotide and three transcribed nucleotides are observed. In the second copy, all four nucleotides are visible ( Supplementary Fig. S2b ). All of the data sets were processed using XDS [32] with XDSAPP GUI [33] . The model building was performed in Coot [34] , and the structures were refined using phenix.refine. The following percentages of the residues were located in the allowed region of the Ramachandran plot: structure (i) −98.7%, structure (ii) −99.8%, and structure (iii) −99.6%. Simulated annealing omit maps were calculated using Phenix, and Pymol was used for structural analyses and the preparation of the structural figures ( http://www.pymol.org ; accessed 1 August 2013). RNA substrate preparation RNA-GG (a 63 nucleotide [nt] RNA oligonucleotide: 5′-GGGTAACGCTATTATTACAAAGCTCTTTTATGTAGTGTGCGTACCACGGTAGCAGGTACTGCG-3′) was produced by in vitro transcription using AmpliScribe T7-Flash Transcription Kit and was subjected to capping reactions using vaccinia virus capping enzymes (Epicentre) [17] . The capping reactions were performed according to the manufacturer’s recommendations with the addition of 10 mCi [α- 32 P] GTP (3,000 Ci mmol −1 ; Hartman Analytic GmbH). Unlabelled substrates were prepared following an analogous procedure with the use of 1 mM guanosine triphosphate instead of its labelled counterpart. The synthesis of m 7 GpppGpApUpC was performed by coupling the 5′-phosphorylated tetranucleotide pGpApUpC (0.5 mg, ammonium salt; TriLink Biotechnologies) with 7-methylguanosine 5′-diphosphate imidazolide (2.7 mg, prepared as described previously [35] ) in 0.2 ml of aqueous 0.2 M N -ethylmorpholine/HCl buffer (pH 7.0) that contained MnSO 4 ·H 2 O (6.4 mg) at room temperature for 24 h. The resulting mixture was subjected to high-performance liquid chromatography preparative purification on an Agilent Technologies 1200 apparatus equipped with a Supelcosil LC-18-T reverse-phase column (4.6 × 250 mm) using a linear gradient of methanol as the mobile phase from 0 to 20% (v/v) in 0.05 M ammonium acetate (pH 5.9) within 15 min at a flow rate of 1 ml min −1 . Ultraviolet detection was performed at 260 nm. The retention times were 10.1 and 10.4 min for the product and substrate, respectively. Appropriate eluates from 10 high-performance liquid chromatography runs were collected and lyophilized to give the product (0.15 mg ammonium salt). The predicted molecular mass for the free acid form is 1,742.0, and the measured mass by high-resolution mass spectrometry (electrospray ionization) was 1,741.3. The synthesized capped tetraribonucleotide was shown to be a substrate for CMTr1 MTase ( Supplementary Fig. S6 ). Methyltransferase assay Methylation reactions with CMTr1 were carried out in 30 mM Tris-HCl (pH 8.4), 150 mM KCl, 1 mM EDTA, 10 mM DTT, 100 mM SAM, 10 U Ribolock with 10 pmol of purified enzyme and 0,25 pmol of substrate RNA in a total volume of 20 μl. The reaction buffer for CMTr2 differed in pH (7.4) and KCl concentration (50 mM). Reactions were carried out for 1 h at 37 °C. BAP protein was used as a negative control. The modified RNA was purified by phenol/chloroform extraction and ethanol precipitation. The RNA was digested with either nuclease P1 (Sigma-Aldrich) or RNase T2 (MoBiTec GmbH). The digestion products were resolved on 21% polyacrylamide/8 M urea gel and visualized by autoradiography (Typhoon Trio, GE Healthcare). Quantitative analysis was performed using ImageQuant software (GE Healthcare). Binding assay Binding reactions with CMTr1 were performed in binding buffer (30 mM Tris-HCl (pH 8.4), 150 mM KCl, 1 mM EDTA, 10 mM DTT, 10 μg ml −1 bovine serum albumin and 10 U Ribolock) with 100 μM SAH, 5 pmol of purified enzyme, 50 fmol of 32 P-labelled substrate RNA and 5 pmol of unlabelled RNA without cap structure (competitor RNA) in a total volume of 20 μl. The reaction buffer for CMTr2 differed with regard to the pH (7.4) and KCl concentration (50 mM). BAP protein was used as a negative control. The reactions were performed for 30 min at 37 °C and filtered through a 0.2 μm nitrocellulose membrane (GE Healthcare) using a Dot-Blot apparatus (Bio-Rad). Each well was washed with 400 μl of the binding buffer. Dried membranes were exposed to a PhosphorImager screen, visualized by autoradiography and quantified using ImageQuant software. Protein and RNA structure prediction and analysis Protein structure prediction, including the identification of structured domains and disordered regions, the prediction of secondary structures and alignment with proteins of known structures, was performed via the GeneSilico web server [36] . Homology modelling of the CMTr2 catalytic domain structure was performed using the FRankenstein’s monster approach [37] , in which a series of starting models based on alternative target-template alignments were generated, and a final hybrid model was constructed by splicing the potentially best folded fragments. For comparative modelling of the conserved core (residues 71–405 of CMTr2), Modeller [38] 9v7 was used. The structure of the terminal regions of the CMTr2 catalytic domain with no clear match to the CMTr1 template (residues 1–70 and 406–423 of CMTr2) was predicted by de novo folding onto the precalculated homology model of the core with constraints on secondary structure using REFINER [39] . Protein three-dimensional model quality throughout the modelling process was assessed by MetaMQAP [22] , a programme that predicts the global accuracy of the protein structural model and deviations of individual residues from the positions of their counterparts in the true (unknown) structure. RNA comparative modelling was performed using ModeRNA [40] , followed by the optimization of local geometry and protein-RNA contacts with the Bio+ version of the CHARMM force field using Hyperchem 8.0 (Hypercube). The mapping of the electrostatic potential on protein surfaces was done with Adaptive Poisson-Boltzmann Solver [41] . The mapping of sequence conservation onto the CMTr1 and CMTr2 catalytic domain structures was done using the ConSurf server [42] with the JTT substitution matrix and Bayesian model for rate inference for the corresponding multiple sequence alignments obtained previously [17] . The multiple sequence alignment and model of the CMTr2 catalytic domain structure were also used to plan site-directed mutagenesis experiments. Structure database searches were performed with DALI. Bacterial overexpression and protein purification Synthetic CMTR1 gene was purchased from imaGenes GmbH (IMAGE ID 4944457) and amplified by PCR using primers that introduced NcoI and XhoI restriction sites that are compatible with the cloning sites of pETMM41 expression vector. After insertion into pETMM41, the CMTR1 gene was flanked on the 5′ end by a sequence that encoded HisTag and MBP. The latter was separated from the CMTR1 gene by a sequence that encoded the tobacco etch virus protease cleavage site. The full-length CMTr1 protein expressed in E . coli was insoluble. For the protein expressed in human embryonic kidney 293 cells, we could not obtain a sufficient amount of material for crystallization; therefore, we decided to work with the isolated RFM domain, which was predicted to be active based on analogous experiments with the Trypanosomal homolog [43] . To determine its boundaries, several N- and C-terminal deletion variants were designed, and constructs based on the pETMM41 expression vector were prepared using the QuikChange kit (Stratagene) or inside-out PCR. Protein variants were overexpressed in the ArcticExpress (DE3) E . coli strain and purified on nickel-charged resin (QIAGEN), and the activity of the soluble truncation variants was tested in the MTase assay (see below). First, we selected a protein variant with a C-terminal deletion of residues 551–835 (CMTr1 1–550 ). It was expressed in E . coli in a soluble form, but it was prone to degradation. We then used CMTr1 1–550 in limited proteolysis experiments that showed that the protein form that was the most stable upon trypsin and chymotrypsin digestion had the same size as the spontaneous degradation product. According to our predictions with the MetaDisorder program [44] , the N-terminus of CMTr1 is rich in intrinsic disorder, which could make it susceptible to spontaneous proteolytic degradation. N-terminal sequencing showed that 125 N-terminal residues were absent. A deletion variant, CMTr1 126–550 , was prepared and overexpressed as a fusion protein with MBP in the ArcticExpress (DE3) E . coli strain (Stratagene). CMTr1 126–550 -MBP expression was induced with 0.3 mM IPTG at an optical density of 0.8, and the cells were further cultured for 24 h at 12 °C. They were next lysed in buffer that contained 100 mM NaCl, 30 mM Tris-HCl (pH 8.5), 10% glycerol, 10 mM β-mercaptoethanol (2-ME), 5 mM imidazole, 1 mg ml −1 lysozyme and a mixture of protease inhibitors. After 30 min, the NaCl concentration was increased to 500 mM. The lysate was sonicated, centrifuged and clarified by filtration. The cleared lysate was then loaded on a 5 ml HisTrap Crude column (GE Healthcare) previously equilibrated with 5 mM imidazole, 500 mM NaCl, 30 mM Tris-HCl (pH 8.5), 10% glycerol and 10 mM 2-ME. CMTr1 126–550 -MBP was eluted in a 40–80 mM imidazole gradient. Selected fractions were dialyzed overnight against a buffer that contained 30 mM NaCl, 30 mM Tris-HCl (pH 8.5), 10% glycerol, 0.5 mM EDTA and 3 mM DTT. After this step, the dialyzed sample was loaded on the MonoQ column (GE Healthcare) previously equilibrated with dialysis buffer. The protein was eluted in a 250–280 mM NaCl gradient and digested overnight at 4 °C using tobacco etch virus protease. The digested sample was loaded on a 5 ml HisTrap Crude column equilibrated with 250–280 mM NaCl, 30 mM Tris-HCl (pH 8.5), 10% glycerol, 0.5 mM EDTA and 3 mM DTT. The flow-through fraction was concentrated and purified on a Superdex 75 10/300GL gel filtration column (GE Healthcare). Selected fractions that contained CMTr1 126–550 were concentrated to 8.5 mg ml −1 and stored at 4 °C in a buffer that contained 100 mM NaCl, 30 mM Tris-HCl (pH 8.5), 10% glycerol, 0.5 mM EDTA and 3 mM DTT. The SeMet derivative of the protein was expressed in minimal medium supplemented with SeMet and purified using the same protocol. Analysis of methylation in vitro with the use of 3 H-methyl-SAM Methylation reactions with CMTr1 were performed in reaction buffer (30 mM Tris-HCl (pH 8.4), 150 mM KCl, 1 mM EDTA, 10 mM DTT and 10 U Ribolock) that contained 1 μCi of [ 3 H-methyl]-SAM, 50 pmoles of substrate and purified enzyme in a total volume of 20 μl. The reaction buffer for CMTr2 differed with regard to pH (7.4) and KCl concentration (50 mM). For CMTr2, the cap01-RNA substrate was used instead of cap0 RNA. After 90-min incubation at 37 °C, the enzyme was heat-denatured at 75 °C for 10 min. The samples were then loaded on DE 81 DEAE paper (Whatmann). Free [ 3 H methyl] SAM was removed by washing the membrane with 50 mM phosphate buffer (pH 7.0). The dried membranes were transferred to scintillation vials with 1 ml of liquid scintillator cocktail (Rotiszint eco plus, Roth). The amount of 3 H-methyl group incorporation into the substrates bound to the membrane was measured using a Tri-Carb 2900 TR Liquid Scintillation Analyzer (Packard Bioscience; Supplementary Figs S5,S6 ). Accession codes : Atomic coordinates and structure factors of CMTr1 crystallographic structures have been deposited in the Protein Data Bank with accession codes 4N48 (complex with m 7 GpppGAUC), 4N49 (complex with m 7 GpppG) and 4N4A (unliganded protein). Atomic coordinates of the CMTr2 model structure are available from http://www.genesilico.pl/iamb/models/RNA.MTases/CMTr2/ and from http://www.figshare.com/articles/Structure_of_CMTr2_in_complex_with_capped_mRNA_theoretical_model/840535 . How to cite this article : Smietanski, M. et al. Structural analysis of human 2′- O -ribose methyltransferases involved in mRNA cap structure formation. Nat. Commun. 5:3004 doi: 10.1038/ncomms4004 (2014).